Dearomatization of aromatic asmic isocyanides to complex cyclohexadienes 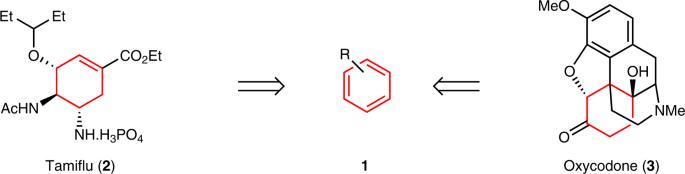Fig. 1: Representative dearomatization-based syntheses. Dearomatizations can rapidly assemble substituted, six-membered rings for the synthesis of bioactive targets such as Tamiflu (2) and Oxycodone (3). A dearomatization-dislocation-coupling cascade rapidly transforms aromatic isocyanides into highly functionalized cyclohexadienes. The facile cascade installs an exceptional degree of molecular complexity: three carbon-carbon bonds, two quaternary stereocenters, and three orthogonal functionalities, a cyclohexadiene, a nitrile, and an isocyanide. The tolerance of arylisocyanides makes the method among the mildest dearomatizations ever reported, typically occurring within minutes at −78 °C. Experimental and computational analyses implicate an electron transfer-initiated mechanism involving an unprecedented isocyanide rearrangement followed by radical-radical anion coupling. The dearomatization is fast, proceeds via a complex cascade mechanism supported by experimental and computational insight, and provides complex, synthetically valuable cyclohexadienes. The dearomatization of substituted arenes is a powerful, complexity-increasing route to diverse carbocycles and heterocycles [1] . Dearomatizations are strategic transformations for assembling complex cyclic, bridged, or spirocyclic scaffolds because multiple bonds are forged from readily available aromatics ( 1 ) [2] , [3] , [4] . Numerous dearomatizations have featured as key steps in the synthesis of prized bioactive targets [5] , [6] , [7] , [8] , [9] where brevity is paramount, such as in the syntheses of the anti-viral drug oseltamivir (Tamiflu, 2 ) [10] and the pain management opiate oxycodone ( 3 ) [11] (Fig. 1 ). Fig. 1: Representative dearomatization-based syntheses. Dearomatizations can rapidly assemble substituted, six-membered rings for the synthesis of bioactive targets such as Tamiflu ( 2 ) and Oxycodone ( 3 ). Full size image The inherent efficiency of dearomatization strategies, the availability of diverse aromatic precursors, and the rapid increase in molecular complexity, have stimulated several creative arene reduction methods [12] . Historically, the advances in dearomatization have followed organic chemistry’s progression from high-energy, two-electron processes (Fig. 2 ) such as dissolving metal reductions ( 1 → 4 ) [13] , carbene ( 5 → 6 ) [14] and organometallic [15] , [16] additions ( 7 → 8 ), and hydrogenation [17] , to more controlled one-electron transfers such as enzymatic ( 1 → 9 ) [18] , oxidative ( 10 → 11 ) [19] , and photochemical ( 1 → 12 ) [20] reactions. Fig. 2: Dearomatization methods: past and present. a Classical dearomatization strategies employing two-electron reductions. b Current dearomatization processes employing one-electron processes. c This SET approach to dearomatization is followed by NC dislocation and radical–radical anion coupling. Full size image This manuscript describes a conceptually unexplored dearomatization strategy employing an organometallic addition to promote a single electron transfer (SET) from an electron-rich aromatic sulfur species to initiate the dearomatization process (Fig. 2 , part c). An SET from an organometallic-activated arylsulfide generates three components from 13 : the isocyanide-stabilized radical 14 , an alkylarylsulfide (ArSR), and the radical anion 15 . Dislocation of the isocyanide within 15 via a formal [3 + 2]-cycloreversion leads to radical anion 16 whose coupling with 14 affords the functionalized cyclohexadiene 17 . The method is possibly the fastest and mildest dearomatization reported, installs an exceptional degree of molecular complexity, and proceeds through an unprecedented dearomatization–dislocation–radical coupling mechanism. Optimization of the dearomatization process Experimental forays to develop the dearomatization method were initiated with the cyclopentylisocyanide 19a , prepared in a single step from the isocyanide building block Asmic ( 18 , Fig. 3 ) [21] . The addition of BuLi to sulfur-substituted isocyanides such as 19a generates electron-rich sulfuranides 20a [22] which, in the presence of TMEDA, intercept electrophiles at the isocyanide-bearing carbon to afford trisubstituted isocyanides such as 21 [21] . Speculating that lithium salts might promote scission of the weak isocyanocarbon–sulfur bond, analogous to halogen–lithium exchange reactions [23] , led to the inclusion of lithium chloride which completely suppressed the formation of 21a ( 21 , R = Bn) to provide 22a in 42% yield (Fig. 3 ); LiBr, LiI, LiOAc, and LiCN were significantly inferior to the use of LiCl. The remarkable formation of 22a reconstitutes the isocyanide 19a both in the aromatic core and the cyclopentylisocyanide. The structural reorganization was confirmed by performing an analogous dearomatization–benzylation of 19a with p -bromobenzyl bromide, initially with LiCl and TMEDA but subsequently in 78% yield with HMTETA in the absence of LiCl (see below), to afford 22b whose structure was unequivocally determined by crystallographic analysis (Fig. 3 ). Fig. 3: Optimization of the dearomatization for isocyanide 19a. Alkylation of Asmic ( 18 ) provides the core scaffold that was dearomatized via sulfuranide 20a to cyclohexadienes 22a and 22b . Full size image Further optimization led to a reappraisal of the role of lithium salts by focusing on complexing agents to change the nature of the sulfuranide 20a . While HMPA and the crown ether Kryptofix 222 proved deleterious, the addition of the TMEDA homolog, PMDTA (pentamethyldiethylenetriamine) [24] afforded 22a in 59% yield. Slow addition of BuLi over 10 min, rather than 30 s, to a solution of 19a and PMDTA provided a small gain to afford 22a in 62% yield. Employing the next highest TMEDA homolog, HMTETA (hexamethyltriethylenetetramine) [25] , afforded 22a with minimal dependence on the addition rate; only one diastereomer was observed in the crude reaction mixture (vide infra). Exploring the scope of the dearomatization The HMTETA-promoted dearomatization protocol provided a rapid route to a range of complex cyclohexadienes (Fig. 4 ). Varying Asmic derivatives were subjected to the dearomatization cascade and trapped with different electrophiles to explore the synthetic potential and substrate scope. Specifically, the use of 19a with allyl bromide or propyl iodide afforded isocyanides 22c and 22d , respectively, with the stereoselective installation of the nitrile-bearing quaternary center as a single diastereomer. Fig. 4: Scope of the dialkylAsmic dearomatization. All yields are of pure, isolated materials following chromatographic purification. Full size image Terminating the dearomatization through protonation or deuteration afforded the 1,3-cyclohexadienes 23a and 23b , consistent with electrophilic trapping of a cyclohexadienylnitrile anion on the γ-carbon [26] . Analogous addition–dearomatization–benzylation sequences were equally efficacious with the 6- and 7-membered Asmic derivatives affording 22e and 22f , respectively. Acyclic Asmic derivatives with methyl, propyl, and hexyl substituents similarly afforded, after benzylation, the corresponding 1,4-cyclohexadienes 22g – 22i ; protonation afforded the 1,3-cyclohexadiene 23c . Diversification in the aromatic ring was explored with Asmic analogs bearing 2-fluorophenyl, 5-chloro-2-methoxyphenyl, and 2, 6-dimethoxyphenylsulfanyl substituents and with two isocyanonaphthylene analogs (Fig. 5 ); an ortho heteroatom appears to be required for the dearomatization as attempts to perform the dearomatization with the p -methoxy analog of 19a cleanly returned unreacted material [27] . A brief optimization with the cyclopentyl- and dipropylfluorophenylisocyanides 24a and 24e identified the TMEDA–LiCl combination as more efficacious than HMTETA; in comparable dearomatizations with 24e , HMTETA afforded 25e in 56% compared to 84% with TMEDA–LiCl. Under optimized conditions, the dearomatization-benzylation afforded the 1,4-cyclohexadiene 25a as a single diastereomer in 82% yield while the analogous allylation afforded 25b . The only significant difference in the reaction of the fluorophenylisocyanides 24 compared with Asmic derivatives 19 (Fig. 4 ) was the need for an extended time for the electrophilic trapping; the fluorine-substituted cyclohexadienyl anion was significantly less nucleophilic than that generated from 19 . Fig. 5: Dearomatization of aryl-substituted dialkylAsmics 24. All yields are of pure, isolated materials following chromatographic purification ( a 1.1 Equiv of HMTETA was used in place of TMEDA and LiCl). Full size image Analogous addition–dearomatization–benzylations with the cyclic 6- and 7-membered fluorophenylisocyanides ( 24b and 24c ) afforded the corresponding cyclohexadienes 25c and 26d , respectively; representative acyclic fluorophenylisocyanides ( 24e – 24g ) afforded 25e – 25g . Extending the sequence to a 5-chloro-2-methoxy-substituted isocyanide ( 24h ) afforded the vinylchloride–vinylether 25h while the dimethoxyphenyl-substituted isocyanide ( 24i ) generated the bis-vinylether 25i in which the congested quaternary center is flanked by two ‘ ortho ’ substituents. Dearomatization of isocyanonaphthalenes proceeded with the same reactivity profile as the phenyl analogs affording 25j for the dearomatization–benzylation, and 25k for the dearomatization-protonation. Computational analysis of the dearomatization mechanism The dearomatization–dislocation–radical coupling sequence is remarkable in installing three different functionalities and two quaternary centers in a single synthetic operation. Early mechanism-driven optimization seemed most consistent with a SET radical process, particularly the sensitivity toward concentration, regioselectivity preferences, the preference for THF as the solvent, and subsequent mechanistic experiments (vide infra). Valuable mechanistic insight was obtained from dispersion-corrected DFT calculations (for representative examples see ref. 28 ) noted as UB3LYP-D3/def2-TZVPP-SMD(THF)//UB3LYP-D3/def2-SVP-SMD(THF) that provided structural information on the role of HMTETA complexes and putative intermediates (Fig. 6 ; the Cartesian coordinates are available in the Supplementary Data file). Fig. 6: Calculated energetics of dearomatization–dislocation-coupling sequence. Free energies (kcal/mol) were computed at the UB3LYP-D3/def2-TZVPP-SMD(THF)//UB3LYP-D3/def2-SVP-SMD(THF) level of theory. Full size image Prior calculations on the sulfur–lithium exchange of dialkylAsmic provided the starting point for computationally probing the influence of chelation [22] . Specifically, the importance of HMTETA to sequester the lithium cation was incorporated into the energetics for the complexation and transfer of the alkyl group from MeLi (as a computational surrogate for BuLi with fewer rotatable bonds) to sulfur (Fig. 6 , A → A ’ ); experimentally, substituting MeLi for BuLi leads to only recovered material without any trace of dearomatization which may be due to complex aggregate equilibria in solution [29] . As shown in Fig. 6 , an initial HMTETA–Li complexation facilitates the methyl transfer from MeLi to sulfur in the dimethylAsmic complex A ’ leading to the formally anionic sulfuranide A0 (in complexation with Li + •••HMTEA) via a low barrier transition state TS0 (barrier ~4.4 kcal/mol from complex A’ ). Lithium complexation appears to prevent heterolytic cleavage of AO to a solvent-separated isocyanide anion, analogous to related lithium complexing agents in similar equilibria [30] . From sulfuranide A0 , concurrent decomplexation and homolytic cleavage of the S-alkyl bond generates the anisole radical anion B •− (akin to those proposed in dissolving metal reductions) and the isocyanide-stabilized radical ( R • ) [31] . Subsequent single electron transfer (SET) from radical anion B •− to dimethylAsmic A [32] , triggers the formation of an alkylarylsulfide B and radical anion A •− calculated to be 2.4 kcal/mol downhill with a SET barrier of 1.0 kcal/mol (see SI) [33] . Experimentally, the isolation of AnSBu in virtually quantitative yield is consistent with the computed conversion of B •− to alkylarylsulfide B . From the key thioaryl radical anion A •− , a facile 5- endo -dig cyclization (only a 6.4 kcal/mol barrier) was found via TS1 to the spirocyclic radical anion C . Subsequent fragmentation of the thiazoline via TS2 completes an unusual isocyanide-to-nitrile dislocation with the release of thioacetone ( D’ ) and formation of radical anion D [34] . 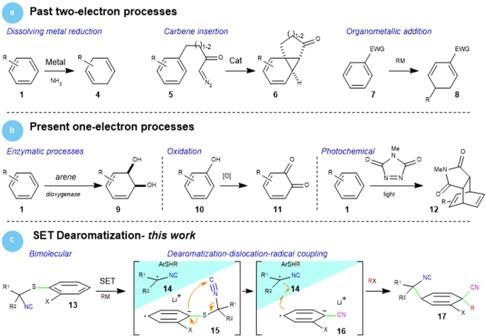Fig. 2: Dearomatization methods: past and present. aClassical dearomatization strategies employing two-electron reductions.bCurrent dearomatization processes employing one-electron processes.cThis SET approach to dearomatization is followed by NC dislocation and radical–radical anion coupling. Consistent with these computations, was the isolation of benzylcyclopentenylsulfide from the putative deprotonation of cyclopentathione followed by trapping with benzyl bromide (see 31 , Fig. 7b ). Fig. 7: DialkylAsmic dearomatization mechanism. a Trapping with diphenylethylene is consistent with the formation of radical intermediates. b The formal [3 + 2] cycloreversion of 28 is consistent with the computationally determined dislocation sequence. Full size image The nitrile-stabilized radical anion D is a persistent anionic radical that has featured in several radical–radical anion couplings [35] , [36] . Radical coupling of D with the isocyanide-stabilized radical R • (from the homolytic cleavage of AO ) affords the highly delocalized dienylnitrile anion E via TS D–E , similar to delocalized anions formed by dissolving metal reduction [26] . The spin density calculations shown in Fig. S3 indicate a higher spin density at the carbon para to nitrile as compared to other positions, which is consistent with the observed coupling regioselectivity [37] . The final bond-forming event, electrophilic trapping of E , is highly diastereoselective, congruent with steric shielding by the isocyanide which directs electrophilic attack to the opposite face via TS3 ; experimentally, the nitrile and isocyanoalkyl substituents are located cis in the cyclohexadiene. Experiments supporting the proposed mechanism Two experiments support the computationally derived mechanism (Fig. 7 ). Performing the dearomatization of 19c and 24f in the presence of the radical trap diphenylethylene in each case afforded the pyrroline 27 , consistent with forming an isocyanide-stabilized radical (Fig. 7a ). Radical capture of diphenylethylene by the isocyanide-stabilized radical 14a to afford 26 followed by cyclization and hydrogen atom abstraction leads to 27 ; no dearomatization was observed. A separate experiment strongly supports the mechanistically reasonable, yet previously unknown, 2,3-type cycloreversion of C via TS2 to D (Fig. 6 ). Sequential exposure of the dihydro-1,3-thiazene 28 to BuLi and BnBr afforded nitrile 30 and vinyl sulfide 31 (Fig. 7b ), paralleling the fragmentation of C to D ; deprotonation of 28 to generate 29 likely triggered cleavage to a metalated nitrile and cyclopentathione whose benzylations led to the benzyl nitrile 30 and the benzyl vinyl sulfide 31 , respectively. The mechanistic insight was invaluable for developing a crossed dearomatization with two different isocyanides, 19c as the SET donor and 24i as the electron acceptor (Fig. 8 ). Addition of BuLi to a mixture of 19c and 24i afforded the cyclohexadiene 25l consistent with preferential complexation of BuLi to the more Lewis basic methoxy group in 19c followed by selective SET to the more electron deficient aromatic 24i . Subsequent fragmentation to the radical anion 16i and coupling with the isocyanide radical 14a , generated from 19c , selectively afforded 25l (Fig. 8 ). The crossed dearomatization of 19c with 24i demonstrates the viability of expanding the dearomatization from a process requiring two equivalents of one isocyanide to a general crossed union of two different components. Fig. 8: Crossed dearomatization with a matched isocyanide pair. Electron-rich 19c serves as the isocyanide donor and the electron-deficient 24i as the aromatic acceptor in forming cyclohexadiene 25l . Full size image The dearomatization–dislocation-coupling of Asmic isocyanides is unprecedented. The dearomatization is among, if not, the fastest dearomatization method known and yet is differentiated from the current suite of dearomatization reactions by tolerating the rather delicate isocyanide functionality. The dearomatizations with isocyanide-containing arenes overcome the difficulty in disrupting the stable aromatic core while maintaining the fragile electronic framework of isocyanides, the precise attribute underlying their exceptional reactivity in multi-component [38] , insertion [39] , addition, and radical reactions [40] , [41] . A series of experimental and computational probes strongly support a unique mechanistic paradigm with the synthetic potential to open rapid routes to highly functionalized scaffolds. 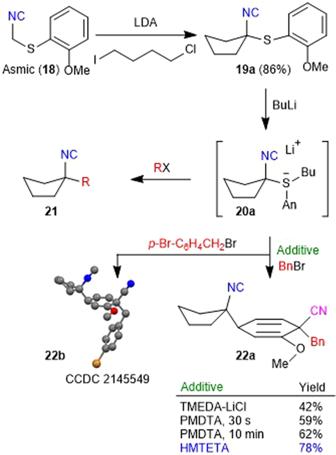Fig. 3: Optimization of the dearomatization for isocyanide 19a. Alkylation of Asmic (18) provides the core scaffold that was dearomatized via sulfuranide20ato cyclohexadienes22aand22b. The dearomatization–dislocation–radical coupling unifies two arylisocyanide components to rapidly assemble a high degree of molecular complexity that forges three carbon–carbon bonds, two quaternary stereocenters, and nitrile and isocyanide functionality in a single operation. The results lay the foundation for exploiting the cascade in expeditiously building complex cyclohexadienes that are inaccessible via current dearomatization methodologies and establishing mechanistic pathways for advancing unexplored bond-forming strategies. Experimental procedures All nonaqueous reactions were performed in flame-dried glassware under a nitrogen atmosphere using Schlenk line techniques. All chemicals were purchased from commercial vendors and used as received unless otherwise specified. Anhydrous tetrahydrofuran (THF) was distilled from benzophenone–sodium under nitrogen before use. Anhydrous HMTETA was prepared by vigorously stirring with CaH 2 under nitrogen for 10 min, allowing the CaH 2 to settle, and then withdrawing the HMTETA from the top of the solution. Anhydrous TMEDA was prepared by vigorous stirring with CaH 2 under nitrogen for 10 min, allowing the CaH 2 to settle, and then withdrawing the TMEDA from the top of the solution. Stock solutions of anhydrous LiCl in anhydrous THF were prepared as follows: LiCl (500 mg) was flame dried under vacuum (heating three times for 2 min each time), allowed to cool to rt, and then sparged with nitrogen (×3). Anhydrous THF (15 mL) was added and then the solution was stirred until the LiCl was completely dissolved to generate a 0.79 M solution. Reactions requiring heating were heated in an oil bath. Reactions were magnetically stirred and monitored by thin layer chromatography (TLC) with glass-backed, 250 µm thickness, F254 hard layer SiliaPlate TLC Plates purchased from Silicycle. 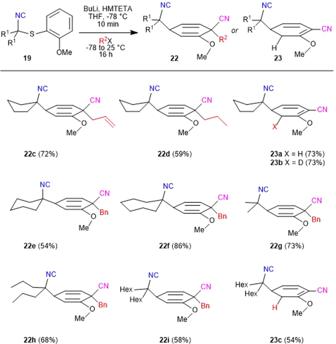Fig. 4: Scope of the dialkylAsmic dearomatization. All yields are of pure, isolated materials following chromatographic purification. TLC plates were visualized using a UV lamp (254 nm) and staining with p -anisaldehyde or potassium permanganate solutions. Flash chromatography was performed with the Buchi Reveleris X2 Automated Flash Chromatography System using SiliaSep™ Flash 40–63 μm, 60 Å silica gel cartridges or manually with SiliaFlash® P60 40–63 μm, 60 Å irregular silica gel purchased from Silicycle. Data analysis 1 H NMR and 13 C{ 1 H} NMR high-resolution nuclear magnetic resonance spectra were recorded on a Varian Mercury Plus 400 (400 MHz/101 MHz) or a Varian Unity Inova 500 (500 MHz/126 MHz) spectrometer at room temperature. Chemical shifts are reported relative to TMS ( δ 0.00) or CDCl 3 ( δ 7.26) for 1 H NMR and CDCl 3 ( δ 77.2) for 13 C{ 1 H} NMR. IR spectra were recorded as thin films (PerkinElmer Spectrum 100 FT-IR Spectrometer). High-resolution mass spectra were obtained on a Thermo-Electron LTQ-FT 7T Fourier transform ion cyclotron resonance (FT-ICR) spectrometer with an atmospheric pressure chemical ionization (APCI) source with direct infusion run in positive ion mode at 5 kV. Additional accurate mass measurement analyses were conducted on either a Waters GCT Premier, time-of-flight, GCMS with electron ionization (EI), or an LCT Premier XE, time-of-flight, LCMS with electrospray ionization (ESI). 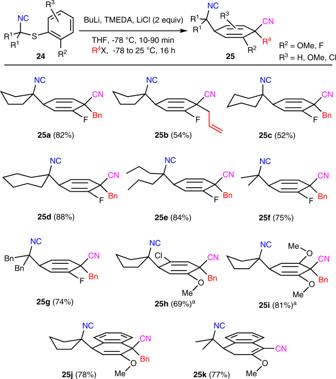Fig. 5: Dearomatization of aryl-substituted dialkylAsmics 24. All yields are of pure, isolated materials following chromatographic purification (a1.1 Equiv of HMTETA was used in place of TMEDA and LiCl). 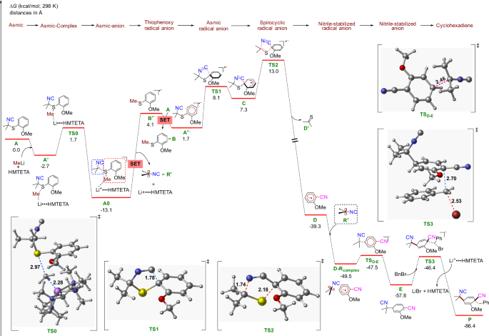Fig. 6: Calculated energetics of dearomatization–dislocation-coupling sequence. Free energies (kcal/mol) were computed at the UB3LYP-D3/def2-TZVPP-SMD(THF)//UB3LYP-D3/def2-SVP-SMD(THF) level of theory. Samples were taken up in a suitable solvent for analysis. The signals were mass measured against an internal lock mass reference of perfluorotributylamine (PFTBA) for EI-GCMS, and leucine enkephalin for ESI–LCMS. Waters software calibrates the instruments, and reports measurements, by use of neutral atomic masses. The mass of the electron is not included. 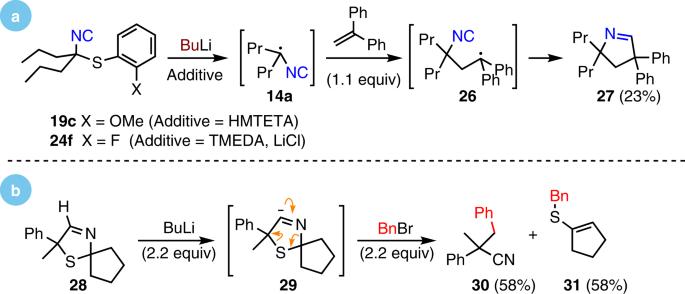Fig. 7: DialkylAsmic dearomatization mechanism. aTrapping with diphenylethylene is consistent with the formation of radical intermediates.bThe formal [3 + 2] cycloreversion of28is consistent with the computationally determined dislocation sequence. 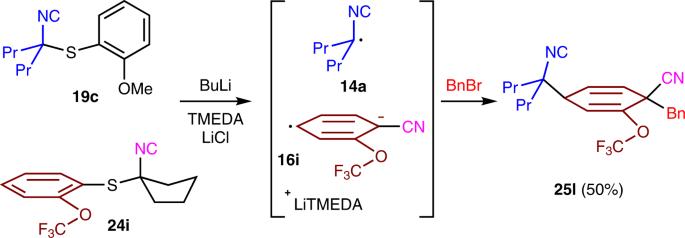Fig. 8: Crossed dearomatization with a matched isocyanide pair. Electron-rich19cserves as the isocyanide donor and the electron-deficient24ias the aromatic acceptor in forming cyclohexadiene25l. Detailed experimental procedures Detailed experimental procedures are provided in the Supplementary Information. Computational analyses Cartesian coordinates of the optimized geometries and vibrational frequencies of the optimized structures are provided in a separate file in the Supplementary Information.